Octapod iron oxide nanoparticles as high-performanceT2contrast agents for magnetic resonance imaging Spherical superparamagnetic iron oxide nanoparticles have been developed as T 2 -negative contrast agents for magnetic resonance imaging in clinical use because of their biocompatibility and ease of synthesis; however, they exhibit relatively low transverse relaxivity. Here we report a new strategy to achieve high transverse relaxivity by controlling the morphology of iron oxide nanoparticles. We successfully fabricate size-controllable octapod iron oxide nanoparticles by introducing chloride anions. The octapod iron oxide nanoparticles (edge length of 30 nm) exhibit an ultrahigh transverse relaxivity value (679.3±30 mM −1 s −1 ), indicating that these octapod iron oxide nanoparticles are much more effective T 2 contrast agents for in vivo imaging and small tumour detection in comparison with conventional iron oxide nanoparticles, which holds great promise for highly sensitive, early stage and accurate detection of cancer in the clinic. Magnetic resonance imaging (MRI) has a critically important role in molecular imaging and clinical diagnosis, because it is non-invasive and is capable of producing images with high spatial and temporal resolution [1] , [2] , [3] . Approximately 35% of clinical MR scans need contrast agents to improve their sensitivity and diagnostic accuracy [4] . For example, superparamagnetic iron oxide nanoparticles are the prevailing T 2 contrast agents, especially for the imaging and detection of lesions in normal tissues [5] , [6] , [7] , [8] . However, there are several challenges for using T 2 contrast agents (for example, Feridex and Resovist) in the clinic. As they are intrinsically negative contrast agents, false-positive diagnosis may be found in the hypointense areas, such as blood pooling, calcification and metal deposition [9] , [10] , [11] . In particular, these commercially available T 2 contrast agents were synthesized in aqueous media and, consequently, exhibit poor crystallinity and relatively low relaxivity [12] . Thus, the primary limitation of MRI is the relatively low sensitivity of the contrast agents [13] , [14] . The development of new T 2 contrast agents with high relaxivity for high-performance MRI diagnosis is required. Considering that the ability of iron oxide nanoparticles for MRI applications is strongly dependent on their sizes and magnetic characteristics, strategies for making iron oxide nanoparticles based on size control and metal doping have been developed [15] , [16] , [17] , [18] . Usually, the larger spherical iron oxide nanoparticles have stronger saturated magnetization ( M s ) and higher T 2 relaxivity ( r 2 ). However, the spherical iron oxide nanoparticles with large size would show ferri/ferromagnetic properties at room temperature, resulting in interparticle agglomeration even in the absence of external magnetic field [12] . On the basis of the quantum mechanical outer sphere theory, the T 2 relaxivity is highly dependent on both the M s value and the effective radius of typically superparamagnetic core [19] , [20] , [21] . In the motional average regime [22] , [23] , the relaxivity r 2 is given by (where all of the nanoparticle contrast agents were simulated as spheres) [24] where M s and r are saturation magnetization and effective radius of magnetic nanostructure, respectively, D is the diffusivity of water molecules, L is the thickness of an impermeable surface coating, and κ is the conversion factor ( κ = V * / C Fe , V * is the volume fraction, C Fe is the concentration of Fe element; for more details, see Supplementary Note 1 ). According to equation (1), we can predict that an increased M s value or larger effective magnetic core radius will result in a higher r 2 value. Although maintaining the M s value (the maximum M s of bulk magnetite is about 92 emu g −1 at room temperature), one can still further achieve a much higher T 2 relaxivity by increasing the effective radius of the magnetic core, which is largely morphology dependent. In the past two decades, controlled synthesis (for example, ion-assisted methods) of unusual and sophisticated metallic nanostructures (for example, octahedral, tetrahexahedral and concave) [25] , [26] , [27] , [28] , [29] is prevailing compared with that of metal oxide nanostructures [30] , [31] , [32] . However, the investigation of iron oxide nanoparticles with different morphologies is rare, probably because it is difficult to prepare iron oxide nanoparticles with diverse shapes. The nanostructure-activity relationship of iron oxide nanoparticles as MRI contrast agents has not been extensively exploited [33] , [34] . Herein, we report a novel strategy to strongly increase T 2 relaxivity by tuning the effective magnetic core radius through morphology control. We successfully synthesize octapod-shaped iron oxide nanoparticles by introducing chloride ions in the reaction system under thermal decomposition conditions. The octapod iron oxide nanoparticles (edge length of 30 nm) exhibit relatively moderate M s (~71 emu g −1 ) but ultrahigh r 2 relaxivity (679.3±30 mM −1 s −1 ) because of the unique structure and highly effective boundary radius. The animal study shows that the octapod iron oxide nanoparticles are suitable as high-performance T 2 contrast agents for in vivo MRI and early tumour detection, particularly for liver lesions. Synthesis and characterization The octapod iron oxide nanoparticles were prepared via decomposition of iron oleate in the presence of sodium chloride (NaCl). Briefly, the iron oleate was decomposed at 320 °C for 2 h in 1-octadecene solvent containing oleic acid as the surfactant and NaCl as the capping agent. Transmission electron microscopy (TEM) images ( Fig. 1a,b ) showed that the as-prepared product consists of uniform four-armed star-like iron oxide particles with high yield (>95%). The average edge length between two nearby armed points is about 30 nm. We observed uniform lattice fringes across the entire nanoparticles with spacing corresponding to Fe 3 O 4 (220) in high-resolution TEM images ( Fig. 1c ). After carefully surveying these unique nanoparticles, we found some shadows likely belong to the four arms of star-like particles, indicating the possible presence of concave feature in the particles. To better visualize the three-dimensional structure of the nanoparticles, we tilted the sample away from the direction perpendicular to the electron beam. Along with the tilting, the nanoparticles changes from four-armed star-like to elongated six-armed stars ( Fig. 1d ), which fits to the feature of octapod nanoparticles owning eight trigonal pyramidal arms [27] . On the basis of these observations, we proposed a concave polyhedral model of this unique iron oxide nanostructure ( Fig. 1a , inset). To confirm this proposed structure, we characterized an individual octapod nanoparticle by high-resolution TEM and relevant selected-area electron diffraction measurements. Both the outlines and angles between the edges of individual nanoparticle are consistent with the geometric models of concave bounded by [311] high-index facets ( Supplementary Fig. S1 ). The X-ray powder diffraction pattern of octapod nanoparticles matched well with magnetite Fe 3 O 4 reference values (JCPDS number 82-1533) without any iron phase, suggesting the octapod iron oxide nanoparticles are pure magnetite with inversed spinel crystal structure ( Supplementary Fig. S2 ). 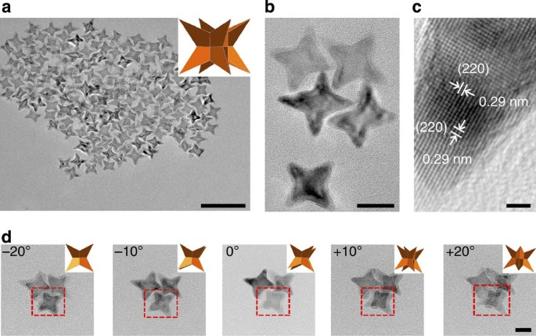Figure 1: TEM analyses of octapod iron oxide nanoparticles. (a) TEM image of Octapod-30 consisted of uniform four-armed star-like particles (inset: geometric model). Scale bar, 100 nm. (b) The higher magnification TEM image of Octapod-30. Scale bar, 20 nm. (c) high-resolution TEM image of Octapod-30, showing the single crystallinity with the lattice fringes across the entire nanoparticles correspond to Fe3O4(220). Scale bar, 2 nm. (d) Tilted TEM images of three Octapod-30. Along with the tilting, the nanoparticles (red dotted squares) change from four-armed star-like to elongated six-armed stars, indicating that the geometric shape of Octapod-30 is a concave octapod owning eight trigonal pyramidal arms (insets: corresponding geometric models). Scale bar, 20 nm. Figure 1: TEM analyses of octapod iron oxide nanoparticles. ( a ) TEM image of Octapod-30 consisted of uniform four-armed star-like particles (inset: geometric model). Scale bar, 100 nm. ( b ) The higher magnification TEM image of Octapod-30. Scale bar, 20 nm. ( c ) high-resolution TEM image of Octapod-30, showing the single crystallinity with the lattice fringes across the entire nanoparticles correspond to Fe 3 O 4 (220). Scale bar, 2 nm. ( d ) Tilted TEM images of three Octapod-30. Along with the tilting, the nanoparticles (red dotted squares) change from four-armed star-like to elongated six-armed stars, indicating that the geometric shape of Octapod-30 is a concave octapod owning eight trigonal pyramidal arms (insets: corresponding geometric models). Scale bar, 20 nm. Full size image Controlled synthesis of octapod iron oxide nanoparticles As expected, NaCl may be essential in the synthesis of octapod iron oxide nanoparticles. We obtained the uniform octapod iron oxide nanoparticles by supplying a certain amount of NaCl (0.17 mmol of NaCl to 0.86 mmol of iron oleate) to a 10 ml of reaction solution. When the amount of NaCl was reduced to 0.085 mmol, the yield of octapod iron oxide nanoparticles was significantly reduced. There were very few octapod iron oxide nanoparticles when the amount of NaCl was further decreased to 0.034 mmol ( Supplementary Fig. S3 ). These results suggest that NaCl may have an important role in the formation of octapod iron oxide nanoparticles. To understand the effects of chloride anions and sodium cations in the formation of octapod iron oxide nanoparticles, we conducted a number of control experiments. When using NaOH and Na oleate instead of NaCl, the products were mainly the mixture of spherical and cubic iron oxide nanoparticles. Similarly, we did not obtain the octapod structure after adding either NaF or KBr in reactions ( Supplementary Fig. S4 ), indicating that the chloride ions are more critical in the formation of octapod iron oxide nanoparticles than of sodium ions. Furthermore, we used hexadecyl trimethyl ammonium chloride, KCl, hexadecyl trimethyl ammonium bromide and KBr instead of NaCl to investigate the structures of final products ( Supplementary Fig. S5 ). The similar octapod products were obtained by adding hexadecyl trimethyl ammonium chloride or KCl, whereas no desired octapod structures were obtained in the presence of hexadecyl trimethyl ammonium bromide or KBr. These results further confirm that the chloride ions are the key inducer of the formation of octapod iron oxide nanoparticles. We were also able to control the sizes of octapod nanoparticles by varying the reaction time in the presence of NaCl. The octapod nanoparticles with average edge lengths of 14, 20, 30 and 36 nm were formed by reaction for 0.5, 1, 2 and 2.5 h, respectively ( Fig. 2a–d ), suggesting that the chloride ions may affect the formation of octapod nanoparticles throughout the particle growth process. One possible mechanism of forming octapod iron oxide nanoparticles was that the chloride ions were selectively bound to iron ions exposed on the high-index facets (probably [311]) of iron oxide during the particle growth ( Fig. 2e,f ). Such a chloride ion-assisted formation mechanism was supported by finding the presence of a trace amount of chlorine on the octapod iron oxide nanoparticles using energy-dispersive X-ray spectroscopy and X-ray photoelectron spectroscopy ( Fig. 2e and Supplementary Fig. S6 ). To the best of our knowledge, this is the first report on the controlled synthesis of unique octapod iron oxide nanostructures with high surface-to-volume ratio ( Supplementary Note 2 ). 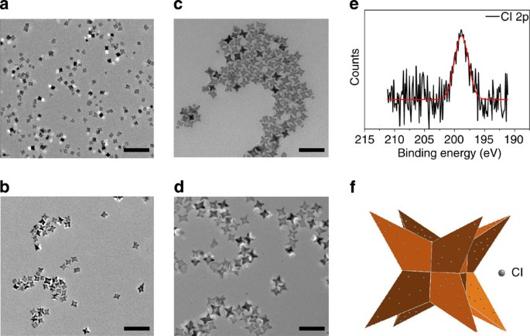Figure 2: Controlled synthesis of octapod iron oxide nanoparticles with different edge lengths. The octapod iron oxide nanoparticles with edge lengths of (a) 14, (b) 20, (c) 30 and (d) 36 nm formed after 1, 1.5, 2 and 2.5 h reaction times in the presence of NaCl, respectively. (e) X-ray photoelectron spectroscopy analysis of octapod iron oxide nanoparticles showed the Cl 2p3/2 peak at 198.9 eV, corresponding to the binding energy of Cl-Fe(III). The red line is a fitted result of the spectrum. (f) The model illustrated that the Cl ions may selectively bind to Fe ions on the surface of octapod iron oxide nanoparticles during size growth. Scale bar, 100 nm. Figure 2: Controlled synthesis of octapod iron oxide nanoparticles with different edge lengths. The octapod iron oxide nanoparticles with edge lengths of ( a ) 14, ( b ) 20, ( c ) 30 and ( d ) 36 nm formed after 1, 1.5, 2 and 2.5 h reaction times in the presence of NaCl, respectively. ( e ) X-ray photoelectron spectroscopy analysis of octapod iron oxide nanoparticles showed the Cl 2p3/2 peak at 198.9 eV, corresponding to the binding energy of Cl-Fe(III). The red line is a fitted result of the spectrum. ( f ) The model illustrated that the Cl ions may selectively bind to Fe ions on the surface of octapod iron oxide nanoparticles during size growth. Scale bar, 100 nm. Full size image Structure and properties of octapod iron oxide nanoparticles Sophisticated morphology of nanostructures may alter the effective radii of particle cores. According to the quantum mechanical outer sphere theory, we simulated a spherical ball covering the full octapod iron oxide nanoparticle as a model to represent the objective existence of octapod nanoparticles under an external magnetic field B 0 ( Fig. 3a ). Thus, the diameter of the model shows the effective diameters of octapod iron oxide nanoparticles. We found the effective radii of octapod iron oxide nanoparticles to be ~2.4 times as large as that of spherical nanoparticles having the same geometric core volumes ( Supplementary Fig. S7 and Supplementary Note 2 ), demonstrating that the octapod morphology can significantly increase the effective radii of nanoparticles and indicating that octapod iron oxide nanoparticles may possess much higher T 2 relaxivity than the spherical nanoparticles with similar geometric volumes. To investigate the MRI contrast ability of octapod and spherical iron oxide nanoparticles with the same geometric volumes, we chose the octapod iron oxide nanoparticles with average edge lengths of 30 nm (denoted as Octapod-30) and 20 nm (denoted as Octapod-20) as two representative examples. Accordingly, spherical nanoparticles with mean diameters of 16 nm (denoted as Spherical-16) and 10 nm (denoted as Spherical-10) were used for comparison because of the similarity in volume (that is, Octapod-30 with Spherical-16 and Octapod-20 with Spherical-10). We then tested the magnetic properties of octapod and spherical iron oxide nanoparticles by a superconducting quantum interference device. Octapod-30, Octapod-20, Spherical-16 and Spherical-10 all showed a smooth M–H curve with no hysteresis at ambient temperature ( Fig. 3b ). The blocking temperature of Octapod-30 and Octapod-20 were 290 K and 240 K, respectively ( Supplementary Fig. S8 ), which further confirmed that Octapod-30 and Octapod-20 exhibited superparamagnetic behaviours at room temperature, enabling these nanoparticles for many biomedical applications (for example, biological separation and MRI contrast enhancement). The M s values of Octapod-30, Octapod-20, Spherical-16 and Spherical-10 were about 71, 51, 67 and 55 emu g −1 , respectively. The slightly higher M s value of Octapod-30 than that of Spherical-16 may be due to the reduced spin canting effect in octapod morphology comparing with spherical particle [35] . Despite of similar M s values, the shape anisotropy in these octapod magnetite nanostructures and significantly increased effective radii of the magnetic cores may be responsible for the distinctly high T 2 relaxivities. 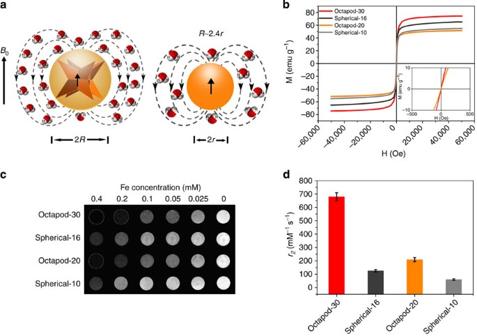Figure 3: MR contrast effect of octapod iron oxide nanoparticles. (a) Schematic cartoon shows the ball models of octapod and spherical iron oxide nanoparticles with the same geometric volume (the black dotted lines represents the magnetic field of the octapod and spherical iron oxide nanoparticles. The same length of black arrow means the sameMsof octapod and spherical iron oxide nanoparticles). With the same geometric core volume, the octapod nanoparticles have much larger effective volume (radius,R) than the spherical nanoparticles (radius,r) withR~2.4runder an external magnetic fieldB0. (b) The smoothM–Hcurves of Octapod-30, Octapod-20, Spherical-16 and Spherical-10 measured at 300 K using a superconducting quantum interference device magnetometer (inset:M–Hcurves of Octapod-30 and Octapod-20 in low-magnetic field areas). TheMsvalues of Octapod-30, Octapod-20, Spherical-16 and Spherical-10 are about 71, 51, 67 and 55 emu g−1, respectively. (c)T2-weigthed MR images of Octapod-30, Octapod-20, Spherical-16 and Spherical-10 in aqueous solution with 1% agarose at various concentrations of iron using a Varian 7T microMRI scanner. (d) Comparison ofr2values of Octapod-30, Octapod-20, Spherical-16 and Spherical-10. The error bars represent ±s.d. of five independent experiments. Figure 3: MR contrast effect of octapod iron oxide nanoparticles. ( a ) Schematic cartoon shows the ball models of octapod and spherical iron oxide nanoparticles with the same geometric volume (the black dotted lines represents the magnetic field of the octapod and spherical iron oxide nanoparticles. The same length of black arrow means the same M s of octapod and spherical iron oxide nanoparticles). With the same geometric core volume, the octapod nanoparticles have much larger effective volume (radius, R ) than the spherical nanoparticles (radius, r ) with R ~2.4 r under an external magnetic field B 0 . ( b ) The smooth M–H curves of Octapod-30, Octapod-20, Spherical-16 and Spherical-10 measured at 300 K using a superconducting quantum interference device magnetometer (inset: M–H curves of Octapod-30 and Octapod-20 in low-magnetic field areas). The M s values of Octapod-30, Octapod-20, Spherical-16 and Spherical-10 are about 71, 51, 67 and 55 emu g −1 , respectively. ( c ) T 2 -weigthed MR images of Octapod-30, Octapod-20, Spherical-16 and Spherical-10 in aqueous solution with 1% agarose at various concentrations of iron using a Varian 7T microMRI scanner. ( d ) Comparison of r 2 values of Octapod-30, Octapod-20, Spherical-16 and Spherical-10. The error bars represent ±s.d. of five independent experiments. Full size image As the as-prepared nanoparticles were hydrophobic and unsuitable for biomedical applications, we transferred the nanoparticles to aqueous media using the conjugates of dendritic molecules and 1-hexadecylamine (denoted as HDA-G 2 ) by a hydrophobic–hydrophobic interaction [36] . The encapsulated nanoparticles showed excellent colloidal stability in aqueous solution. We did not observe any aggregations or morphology alteration after storage for more than 1 month ( Supplementary Fig. S9 ). Furthermore, we measured the hydrodynamic diameters (HDs) of all the samples by dynamic light scattering. The HDs of Spherical-10, Spherical-16, Octapod-20 and Octapod-30 were 22±2, 30±3, 49±5 and 58±2 nm, respectively ( Supplementary Fig. S9 ), suggesting that the iron oxide nanoparticles were monodisperse in water without any clustering and aggregation. Moreover, there are a large number of free amine groups available on the surface of the water-dispersible octapod nanoparticles, allowing for further modification and functionalization. It is of note that the HD of Octapod-30 is about twice as much as that of Spherical-16, which is consistent with the proposed model ( Fig. 3a ). In addition, the physical surface-to-volume ratio of Octapod-30 in aqueous medium is larger than that of the simulated spherical model because of the unique octapod structure. Hence, it is expected that the effective surface area of Octapod-30 for diffusion of water molecules may be more than four times greater than that of Spherical-16. Transverse relaxivity of octapod iron oxide nanoparticles We then tested the transverse relaxivity ( r 2 ) values of the above four samples by a 7T MR scanner. With the increase of Fe concentrations, the signal intensity of T 2 -weighted phantom images obviously decreased ( Fig. 3c ), indicating that all the samples have the potential to generate MRI contrast enhancement on T 2 -weighted sequences. Notably, the octapod iron oxide nanoparticles exhibited stronger T 2 contrast effects than spherical iron oxide nanoparticles, suggesting that the octapod iron oxide nanoparticles may serve as highly sensitive T 2 contrast agents. The r 2 values of Octapod-30, Octapod-20, Spherical-16 and Spherical-10 were about 679.25±30, 209.03±15, 125.86±9 and 59.91±6 mM −1 s −1 , respectively ( Fig. 3d and Supplementary Figs S10 and S11 ). Because of the increased effective radii of octapod iron oxide cores, the r 2 value of Octapod-30 was ~5.4 times larger than that of Spherical-16. Meanwhile, Octapod-20 has a higher r 2 value than Spherical-10 (about 3.5 times) as well. It should be mentioned that the M s values and geometric volumes of both octapod iron oxide nanoparticles were very close to the corresponding spherical iron oxide nanoparticles (that is, Octapod-30 to Spherical-16 and Octapod-20 to Spherical-10). Our results demonstrate that structurally increasing the effective radii of iron oxide through morphology control is an attractive alternative to existing strategies, such as metal doping and particle clustering [18] , [37] , [38] , [39] to increase the T 2 relaxivity of iron oxide nanoparticles. Liver MRI using octapod iron oxide nanoparticles Iron oxide nanoparticles as T 2 contrast agents have been extensively used in liver MRI. Before the animal study, we first tested the cytotoxicity of water-dispersible octapod iron oxide nanoparticles using HepG2 cell line as a model. The MTT (3-(4,5-dimethylthiazol-2-yl)-2,5-diphenyltetrazolium bromide) assay indicated that octapod iron oxide nanoparticles have no appreciable cytotoxicity for 24 h even at concentration up to 100 μg Fe per ml, suggesting the high biocompatibility of the octapod iron oxide nanoparticles ( Supplementary Fig. S12 ). To verify that octapod iron oxide nanoparticles display better contrast effects than traditional spherical iron oxide nanoparticles in vivo , we chose Octapod-30 and Spherical-16 as representative samples and conducted T 2 -weigthed MRI of liver using BALB/c mouse as a model. After intravenous injection of Octapod-30 and Spherical-16 samples at a dose of 1 mg Fe per kg of mouse body weight, we indeed observed significant signal attenuation in the liver region for both nanoparticles ( Fig. 4a ) at 0.5 h post injection (p.i.). To quantify the contrast, we identified the liver as the region of interest and calculated the signal-to-noise ratio (SNR) and SNR post /SNR pre value for each animal ( Fig. 4b and Supplementary Table S1 ). It appears that the Octapod-30 exhibited much higher contrast (63.9±3.2 and 67.3±1.3% at 0.5 and 1 h p.i., respectively) than Spherical-16 (39.8±1.5 and 53.5±1.6% at 0.5 and 1 h p.i., respectively), suggesting that Octapod-30 with higher r 2 value is more sensitive than Spherical-16 in T 2 imaging of liver in vivo . Prussian blue staining detected blue spots throughout the liver sections after administration of Octapod-30 and Spherical-16 ( Supplementary Fig. S13 ), confirming that the signal attenuation in the liver was caused by iron oxide nanoparticle accumulation. The inductively coupled plasma mass spectrometry analysis ( Supplementary Fig. S14 ) indicates that the liver uptake of Octapod-30 and Spherical-16 is in a comparable manner, demonstrating that the much better contrast is due to the higher r 2 value of Octapod-30. In MRI, lower dose of contrast agents may imply lower cost and less side effect, which pledges greater prospects in clinical diagnosis. The high contrast of Octapod-30 prompted us to conduct liver MRI at a lower dose. By reducing the injection dose of Octapod-30 to 0.5 mg Fe per kg, the contrast (39.9±2.5% at 0.5 h and 56.2±1.9% at 1 h) was still slightly higher than that when Spherical-16 at 1 mg kg −1 does ( Supplementary Fig. S15 and Supplementary Table S1 ). 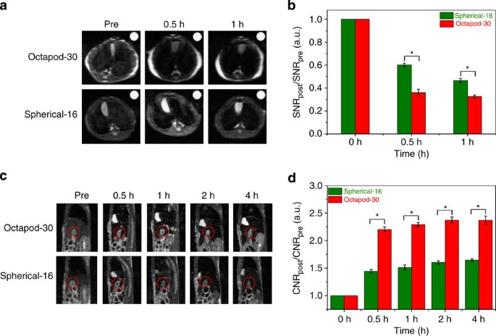Figure 4:In vivMRI. (a)In vivoMR images of BALB/c mice at 0, 0.5 and 1 h after intravenous injection of Octapod-30 (upper) and Spherical-16 (lower) in transverse plane, respectively (the white dot is the signal reference using water in an NMR tube). (b) Quantification of liver contrast collected at 0, 0.5 and 1 h after accumulation of Octapod-30 and Spherical-16 in BALB/c mice at dose of 1.0 mg Fe per kg, respectively (*P<0.01). (c)In vivoMR images of orthotopic xenograft liver tumour model at 0, 0.5, 1, 2 and 4 h after intravenous injection of Octapod-30 and Spherical-16 in sagittal plane. (d) Quantification of contrast-to-noise ratio (CNR) of tumour-to-liver contrast at 0, 0.5, 1, 2 and 4 h after administration of Octapod-30 and Spherical-16, with a dose of 2.0 mg Fe per kg, respectively (*P<0.01). Figure 4: In viv MRI. ( a ) In vivo MR images of BALB/c mice at 0, 0.5 and 1 h after intravenous injection of Octapod-30 (upper) and Spherical-16 (lower) in transverse plane, respectively (the white dot is the signal reference using water in an NMR tube). ( b ) Quantification of liver contrast collected at 0, 0.5 and 1 h after accumulation of Octapod-30 and Spherical-16 in BALB/c mice at dose of 1.0 mg Fe per kg, respectively (* P <0.01). ( c ) In vivo MR images of orthotopic xenograft liver tumour model at 0, 0.5, 1, 2 and 4 h after intravenous injection of Octapod-30 and Spherical-16 in sagittal plane. ( d ) Quantification of contrast-to-noise ratio (CNR) of tumour-to-liver contrast at 0, 0.5, 1, 2 and 4 h after administration of Octapod-30 and Spherical-16, with a dose of 2.0 mg Fe per kg, respectively (* P <0.01). Full size image Detection of liver cancer by MRI To further evaluate the ability of Octapod-30 for liver cancer imaging, we conducted a T 2 -weigthted MRI on an orthotopic HepG2 tumour model. We established the orthotopic liver tumour model by inoculation of small subcutaneous HepG2 tumour fragments into the liver of nude mice. When the hepatic carcinoma reached 3–5 mm in diameter, we intravenously injected Octapod-30 and Spherical-16 into the nude mice (2 mg Fe per kg) and scanned the animals at a 7T microMRI scanner. As hepatic tumours contain much less active Kupffer cells and macrophages [36] , they do not accumulate iron oxide nanoparticles as efficiently as normal liver tissues do [40] , [41] . Thus, the hepatic tumours would show pseudo-positive contrast as compared with normal liver tissues. Both particles caused obvious contrast enhancement in the tumour sites after intravenous administration ( Fig. 4c ). Moreover, the injection of Octapod-30 resulted in higher MR contrast in the tumour site than Spherical-16, leading to easy differentiation between the liver lesions and normal liver tissues in the MR images. The tumour-to-liver contrast increased over time and was as high as 136.9±8.5 and 64.5±2.7% at 4 h p.i. for Octapod-30 and Spherical-16, respectively ( Fig. 4d and Supplementary Table S2 ), indicating that Octapod-30 exhibited much higher signal changes for liver tumour imaging and detection limit than Spherical-16. The use of Octapod-30 with ultrahigh T 2 relaxivity as contrast agent may significantly improve the sensitivity of T 2 imaging, which should be extremely important for accurate detection and early diagnosis of cancer. We further compared the r 2 values of spherical nanoparticles with mean diameter of 25 nm (donated as Spherical-25) and Octapod-20, which have the similar effective diameters (HDs). The results demonstrated that the r 2 value of Octapod-20 is somewhat higher than that of Spherical-25, although the M s value of Spherical-25 is larger than that of Octapod-20 ( Supplementary Fig. S11 ). This phenomenon may be attributed to the strong inhomogeneity of the local magnetic fields induced by the unique octapod-shaped iron oxide nanoparticles, suggesting that the outer sphere theory may have limitations when applied to nanoparticles with significant anisotropy [21] . Because of the unique morphology of octapod iron oxide nanoparticles, the local magnetic field induced by an octapod iron oxide nanoparticle under an external magnetic field ( B 0 ) may be more inhomogeneous than that of a spherical one, which may further induce proton dephasing and enhance the T 2 shortening [42] . On the basis of the calculations using the Landau–Lifshitz–Gilbert equation, we found that the octapod morphology did result in a significantly more inhomogeneous induced magnetic field than the spherical one as expected, whereas the induced magnetic field in the far field (micrometer away) is negligible (~10 −3 Oe) and almost the same regardless of the nanoparticle shape ( Supplementary Fig. S16 and Supplementary Table S3 ). These results indicate that octapod iron oxide nanoparticles could further increase the r 2 value by inducing a more inhomogeneous magnetic field. The fact that the r 2 value of Spherical-25 is close to that of Octapod-20 manifests that the increased effective radius is the main reason to improve the transverse relaxivity of octapod iron oxide nanoparticles. In summary, we have demonstrated a novel strategy for designing concave octapod iron oxide nanoparticles with ultrahigh r 2 values as T 2 contrast agents. The key to successful fabrication of size-controllable octapod iron oxide nanoparticles is the presence of chloride anions. It turns out that by increasing the effective radius and local field inhomogeneity of the magnetic core, the octapod iron oxide nanoparticles exhibit an incredibly high T 2 contrast enhancement effect. The controlled synthesis of octapod iron oxide nanoparticles is facile, highly reproducible and amenable to scale up, thereby rendering these novel iron oxide nanoparticles promising T 2 contrast agents for MRI. This new strategy of achieving extremely high T 2 relaxivity of iron oxide nanoparticles by increasing the effective radii of iron oxide cores rather than the magnetization values is believed to be critically important in developing highly sensitive second-generation contrast agents for MRI ( Supplementary Table S4 ), especially for the early and accurate diagnosis of liver cancer in patients. Moreover, the controllable synthesis of novel octapod iron oxide nanoparticles, together with other morphologies (for example, sphere, cube and rod), certainly facilitates the applications of magnetic nanoparticles in high-density data storage, hyperthermia treatment and magnetically guided drug delivery. Synthesis of octapod iron oxide nanoparticles In a typical synthesis of octapod iron oxide nanoparticles, iron oleate (0.8 g, 0.86 mmol), NaCl (10 mg, 0.17 mmol), oleic acid (110 μl, 0.35 mmol) and distilled water (60 μl) were mixed together with 10 ml of 1-octadecene. The resulting solution was degassed in vacuum for 30 min and backfilled with argon to remove any low volatile impurities and oxygen at room temperature. And then, we heated the reaction solution to 320 °C with a constant heating rate of 3.3 °C min −1 , and were kept at the temperature for 2 h. The colour of the solution changed from reddish-brown to transparent orange and finally brownish-black. Then, the solution was cooled to room temperature and mixed with 30 ml of isopropanol to precipitate the nanoparticles. The nanoparticles were separated by centrifugation and washed three times with ethanol. The final product was dissolved in hexane for long-term storage at 4 °C. See Supplementary Methods for further details of synthesis procedures. Measurement of T 2 relaxivities To measure the T 2 relaxivity, Octapod-30, Octapod-20, Spherical-16 and Spherical-10 with different iron concentrations were dispersed in 1% agarose solution. The samples were scanned (at 300 K) using a T 2 -weighted fast spin-echo multi-slice sequence (fSEMS) (TR/TE=2,000/20, 40, 60, 80, 100 ms, slice thickness=2 mm) by a 7T MRI scanner (Varian 7T microMRI System). In vivo liver MRI Animal experiments were executed according to the protocol approved by Institutional Animal Care and Use Committee of Xiamen University. We performed the in vivo MRI of liver by using BALB/c mouse as a model. After intravenous injection of iron oxide nanoparticles at a dose of 1 mg Fe per kg of mouse body weight, the coronal and transverse plane MR images were scanned using an fSEMS (TR/TE=3,000/40 ms, 256 × 256 matrices, averages=1) on a Varian 7T microMRI scanner. The MR images were obtained at pre-injection, 0.5 and 1 h p.i. ( n= 3 per group). To qualify the signal enhancement, we calculated the SNR by the equation: SNR liver =SI liver /SD noise , where SI represents signal intensity and SD represents s.d. In vivo liver tumour imaging We established the orthotopic liver tumour model by inoculation of small subcutaneous HepG2 tumour fragments into the liver of nude mice. When the tumour reached 3–5 mm in diameter, mice were intravenously injected with Octapod-30 and Spherical-16 at a dose of 2 mg Fe per kg. The coronal and transverse plane MR images were acquired using an fSEMS (TR/TE=3,000/40 ms, 256 × 256 matrices, averages=1) on a 7T MRI scanner. The MR images were sequentially obtained at 0, 0.5, 1, 2 and 4 h p.i. ( n= 3 per group). To qualify the efficacy of contrast enhancement, we introduced the CNR (contrast-to-noise ratio), which was given by CNR=(SNR tumour –SNR liver )/SNR tumour . How to cite this article: Zhao, Z. et al. Octapod iron oxide nanoparticles as high-performance T 2 contrast agents for magnetic resonance imaging. Nat. Commun. 4:2266 doi: 10.1038/ncomms3266 (2013).